Behavioural memory reconsolidation of food and fear memories The reactivation of a memory through retrieval can render it subject to disruption or modification through the process of memory reconsolidation. In both humans and rodents, briefly reactivating a fear memory results in effective erasure by subsequent extinction training. Here we show that a similar strategy is equally effective in the disruption of appetitive pavlovian cue–food memories. However, systemic administration of the NMDA receptor partial agonist D-cycloserine, under the same behavioural conditions, did not potentiate appetitive memory extinction, suggesting that reactivation does not enhance subsequent extinction learning. To confirm that reactivation followed by extinction reflects a behavioural analogue of memory reconsolidation, we show that prevention of contextual fear memory reactivation by the L-type voltage-gated calcium channel blocker nimodipine interferes with the amnestic outcome. Therefore, the reconsolidation process can be manipulated behaviourally to disrupt both aversive and appetitive memories. The retrieval of an established memory is not a passive process. Memory retrieval has long been recognized as an active constructive process [1] , and is more recently thought of as a means of memory modification [2] . Under certain circumstances, memory retrieval 'reactivates' the memory, destabilizing it and engaging a process of post-retrieval plasticity that is known as memory reconsolidation. The long-lasting amnesia that results from disruption of memory reconsolidation has canonically been achieved using cellular or pharmacological interventions in models of pavlovian fear conditioning in both rodents and humans [3] , [4] , but also in preclinical models of reward-seeking behaviour [5] , [6] . These findings have raised the prospect of reconsolidation-based therapeutic interventions for conditions such as post-traumatic stress disorder [7] and drug addiction [8] . Recently, a purely behavioural analogue of pharmacologically induced reconsolidation impairments has been developed, making use of reactivation-induced memory plasticity to diminish pavlovian fear memories through non-reinforced stimulus exposure. In both rodents and humans, this combination of reactivation-induced reconsolidation and behavioural extinction training has resulted in a reduction of fear memory expression that does not recover with normally effective reminder procedures [9] , [10] , [11] . The potential translational efficacy of this approach remains unclear, especially given some noted failures to replicate the effects [12] , [13] . Moreover, there is also the question of its relevance to appetitive reward-related memories. The association of a conditioned stimulus (CS) with a rewarding outcome results in long-lasting conditioned reinforcing properties that powerfully influence reward-seeking behaviour [14] . We have previously shown that the CS–reward memories supporting conditioned reinforcement undergo reconsolidation for both sucrose and cocaine rewards [5] , [6] , [15] , and that disruptive effects in this procedure are reliably predictive of impairments in other translationally relevant models of reward-seeking behaviour [16] , [17] , [18] . Here we also show that the behavioural approach of combining memory reactivation with extinction training is effective in disrupting appetitive pavlovian memories. The amnestic effect of extinguishing a reactivated memory has been interpreted within the framework of memory reconsolidation [9] , [10] , [11] . However, it is equally plausible that prior memory reactivation may potentiate subsequent extinction in a similar manner to pharmacological enhancement of extinction. Treatment with the NMDA receptor partial agonist D-cycloserine (DCS) or Fibroblast growth factor 2 enhances fear memory extinction [19] , [20] , [21] . Importantly, this potentiated memory extinction is not subject to normal recovery, suggesting that extinction enhancement can lead to the same qualitative outcome as reconsolidation impairment. We sought to disambiguate these accounts by selectively disrupting memory reactivation. Contextual fear memory destabilization on reactivation depends on calcium influx at L-type voltage-gated calcium channels (LVGCCs), as shown by the effect of the LVGCC blocker nimodipine to protect against the amnestic effect of protein synthesis inhibition [22] . Therefore, we show first that memory reactivation and extinction impairs contextual fear memories, and, subsequently, that this effect depends critically on LVGCC-mediated memory reactivation. Appetitive pavlovian memory First, we tested the effect of combining a brief memory reactivation and, at an interval of 1 h, as demonstrated to be effective in a fear memory paradigm [9] , a longer memory extinction session on an appetitive pavlovian light–food memory. This was conducted in a procedure that isolates the acquired pavlovian conditioned reinforcing properties of appetitive conditioned stimuli, tested through the acquisition of discriminated lever pressing for the CS. We selected such a procedure as it is acutely sensitive to disruption of the pavlovian memory, and we have previously used it to demonstrate reconsolidation impairments for both sucrose– and cocaine–associated memories [5] , [6] , [15] . Moreover, disruptive effects in this procedure are reliably predictive of impairments in other translationally relevant models of reward-seeking behaviour [16] , [17] , [18] . An overall mixed ANOVA of all the experimental conditions described below revealed significant lever × group ( F (5,42)=3.681, P =0.007) and lever × session × group ( F (18.3,154.1)=2.130, P =0.007) interactions, as well as a main effect of group ( F (5,42)=4.050, P =0.004). This indicates that the groups differed in their acquisition of discriminated responding over the multiple testing sessions. To explore this overall effect, we first analysed the simple session × group interactions for the active and inactive levers independently (mixed ANOVA, P <0.025, using Bonferroni correction for multiple comparisons). For the active lever, there was both a session × group interaction ( F (16.5,138.3)=2.316, P =0.004) and a significant effect of group ( F (5,42)=4.117, P =0.004). In contrast, there were no group differences on responding on the inactive lever (session × group: F (19.0,159.9)=1.166, P =0.293; group: F (5,42)=2.619, P =0.038). Given the selective effect on the active lever response rates, post-hoc pairwise comparisons (mixed ANOVA, P <0.01, using Bonferroni correction) were conducted between each experimental group and the control extinction-alone group that received all 70 min of extinction training in a single session. Firstly, the combination of reactivation and extinction (reactivation+extinction) resulted in a marked and persistent reduction in conditioned reinforcement ( Fig. 1a,b ; session × group: F (2.5,29.7)=2.010, P =0.43; group: F (1,12)=10.045, P =0.008). This disruption was observed through 6 test sessions over 20 days following reactivation and extinction. Moreover, no recovery was seen here in a reinstatement test on day 27. Therefore, there was no evidence of recovery from the memory deficit induced by reactivation + extinction. Similar to fear memories [9] , there was a critical temporal window following memory reactivation, during which the extinction session must be applied to produce the amnestic effect. Delaying extinction to 6 h after reactivation resulted in acquisition of active lever responding that was not different from the control extinction group ( Fig. 1c ; session × group: F (1.9,24.6)=0.532, P =0.584; group: F (1,13)=3.653, P =0.078). 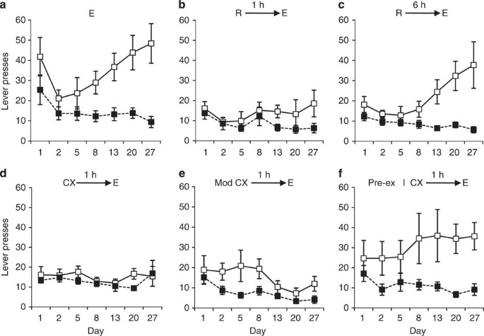Figure 1: Acquisition of a new response with conditioned reinforcement. Discriminated responding on the active (open symbols) and inactive (filled symbols) levers was compared across experimental conditions. (a) Extinction (E) alone, without prior memory reactivation (N=7). (b) Reactivation (R) followed, 1 h later, by extinction (N=7). (c) Reactivation followed, 6 h later, by extinction (N=8). (d) Context exposure (CX) followed, 1 h later, by extinction (N=12). (e) Exposure to modified (Mod) context followed, 1 h later, by extinction (N=7). (f) Pre-training context habituation (pre-ex), with post-training context exposure followed, 1 h later, by extinction (N=7). Groups b, d & e differed significantly from the control group a. Groups c & f did not differ from group a. Data presented as mean±s.e.m. Figure 1: Acquisition of a new response with conditioned reinforcement. Discriminated responding on the active (open symbols) and inactive (filled symbols) levers was compared across experimental conditions. ( a ) Extinction (E) alone, without prior memory reactivation ( N =7). ( b ) Reactivation (R) followed, 1 h later, by extinction ( N =7). ( c ) Reactivation followed, 6 h later, by extinction ( N =8). ( d ) Context exposure (CX) followed, 1 h later, by extinction ( N =12). ( e ) Exposure to modified (Mod) context followed, 1 h later, by extinction ( N =7). ( f ) Pre-training context habituation (pre-ex), with post-training context exposure followed, 1 h later, by extinction ( N =7). Groups b, d & e differed significantly from the control group a. Groups c & f did not differ from group a. Data presented as mean±s.e.m. Full size image In a finding notably different from fear memories [9] , when memory reactivation was replaced by a session in which the rats were simply returned to the experimental context for 10 min without exposure to the light CS (that is, the nosepoke response had no consequence), its combination with extinction 1 h later still produced a marked deficit in conditioned reinforcement compared with the extinction controls ( Fig. 1d ; session × group: F (2.3,39.7)=3.827, P =0.025; group: F (1,17)=17.299, P =0.001). One likely explanation for the capacity of context exposure alone to reactivate the light–food memory in the current study is that the context acts as an occasion-setting stimulus. In this procedure, the context is consistently associated with the light–food memory over 9 days of training, whereas fear conditioning takes place over a single short training session. Alternatively, it is possible that the instrumental setting of the procedure results in nosepoke responding during the context exposure session being sufficient to retrieve and reactivate the CS–food association even in the absence of explicit CS exposure. The latter explanation is rendered less likely by the observation that preventing the nosepoke response during context exposure failed to mitigate the deficit in conditioned reinforcement ( Fig. 1e ; session × group: F (2.3,27.9)=5.026, P =0.011; group: F (1,12)=10.152, P =0.008). Instead, when rats were pre-exposed to the context for 3 h over 2 days before training, context exposure no longer reactivated the memory sufficiently to induce a subsequent deficit in conditioned reinforcement ( Fig. 1f ; session × group: F (2.5,29.4)=1.196, P =0.323; group: F (1,12)=0.288, P =0.601). This indicates that context pre-exposure resulted in habituation to the context, slowing or preventing the acquisition of any contextual modulatory impact during training, and hence reduced the capacity of post-training context exposure to reactivate the CS–food memory. None of the previously described behavioural effects during the test sessions was easily attributable to prior differences in training history other than the experimental manipulations. The total number of CS–food pairings did not differ between the groups ( Fig. 2a ; one-way ANOVA; F (5,42)=0.605, P =0.697). Similarly, there was no difference in the number of unreinforced CS presentations during memory reactivation ( Fig. 2b ; one-way ANOVA; F (2,19)=0.162, P =0.852) or extinction ( Fig. 2c ; one-way ANOVA; F (5,42)=1.446, P =0.228). Therefore, there is no pattern of differences during training and reactivation/extinction that can account for the observed selective disruption of conditioned reinforcement. 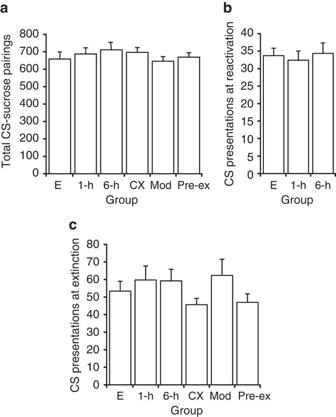Figure 2: No differences between groups before acquisition of a new response with conditioned reinforcement. The groups were extinction alone (E;N=7); reactivation + extinction with a 1-h interval (1-h; N=7); reactivation + extinction with a 6-h interval (6-h,N=8); context exposure followed by extinction (CX;N=12); exposure to modified context before extinction (mod;N=7) and pre-exposure to the context before training (pre-ex;N=7). (a) Total number of CS–sucrose pairings during training across all groups. (b) Number of unreinforced CS presentations during memory reactivation in groups 1-h and 6-h compared with the equivalent first 10 min of extinction in group E. (c) Number of unreinforced CS presentations during memory extinction across all groups compared with the equivalent final 60 min of extinction in group E. Data presented as mean+s.e.m. Figure 2: No differences between groups before acquisition of a new response with conditioned reinforcement. The groups were extinction alone (E; N =7); reactivation + extinction with a 1-h interval (1-h; N=7); reactivation + extinction with a 6-h interval (6-h, N =8); context exposure followed by extinction (CX; N =12); exposure to modified context before extinction (mod; N =7) and pre-exposure to the context before training (pre-ex; N =7). ( a ) Total number of CS–sucrose pairings during training across all groups. ( b ) Number of unreinforced CS presentations during memory reactivation in groups 1-h and 6-h compared with the equivalent first 10 min of extinction in group E. ( c ) Number of unreinforced CS presentations during memory extinction across all groups compared with the equivalent final 60 min of extinction in group E. Data presented as mean+s.e.m. Full size image When rats were injected with DCS, instead of being reactivated, before the 1-hr memory extinction session, there was no effect on subsequent acquisition of the new response with conditioned reinforcement. Rats injected with DCS and saline did not differ in lever pressing ( Fig. 3a,b ; mixed ANOVA; lever × group: F (1,13)=0.004, P =0.949; lever × session × group: F (2.0,25.8)=0.345, P =0.710; group: F (1,13)=0.420, P =0.528), with both groups showing the acquisition of discriminated lever pressing over the course of testing (lever: F (1,13)=19.800, P =0.001; lever × session: F (2.0, 25.8)=8.750, P =0.001). Neither group differed during training or extinction, receiving both similar total numbers of light–food pairings (Saline=581.5±28.1, DCS=609.9±29.4; one-way ANOVA; F (1,13)=0.478, P =0.501) and similar numbers of non-reinforced light presentations during extinction (Saline=63.0±5.8, DCS=66.6±8.6; one-way ANOVA; F (1,13)=1.297, P =0.275). 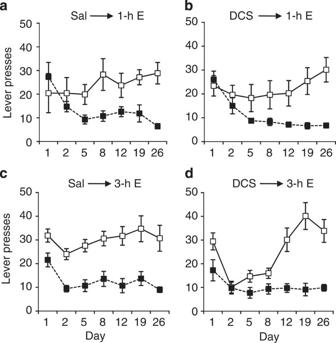Figure 3: D-cycloserine potentiates extinction when the extinction session is 3-h but not 1-h long. Discriminated responding on the active (open symbols) and inactive (filled symbols) levers was compared across experimental conditions. (a) Saline injection before 1-h extinction (N=7). (b) DCS injection before 1-h extinction (N=8). (c) Saline injection before 3-h extinction (N=7). (d) DCS injection before 3-h extinction (N=8). DCS had no effect on the acquisition of discriminated responding with conditioned reinforcement with the 1-h extinction session, but did retard acquisition with the 3-h session. Data presented as mean±s.e.m. Figure 3: D-cycloserine potentiates extinction when the extinction session is 3-h but not 1-h long. Discriminated responding on the active (open symbols) and inactive (filled symbols) levers was compared across experimental conditions. ( a ) Saline injection before 1-h extinction ( N =7). ( b ) DCS injection before 1-h extinction (N=8). ( c ) Saline injection before 3-h extinction ( N =7). ( d ) DCS injection before 3-h extinction ( N =8). DCS had no effect on the acquisition of discriminated responding with conditioned reinforcement with the 1-h extinction session, but did retard acquisition with the 3-h session. Data presented as mean±s.e.m. Full size image The functional effect of DCS to potentiate memory extinction was confirmed in the present appetitive setting when a longer 3-h extinction session was used ( Fig. 3c,d ). Rats injected with DCS and saline differed in lever pressing (mixed ANOVA; lever × session × group: F (3.4,40.6)=3.129, P =0.031; lever × group: F (1,12)=1.757, P =0.210; group: F (1,12)=3.176, P =0.100). Analysis of simple effects of group and session by mixed ANOVA revealed a significant effect of DCS on responding on the active (session × group: F (3.0,36.4)=3.404, P =0.027; group: F (1,12)=4.462, P =0.056), but not the inactive lever (session × group: F (3.1,36.8)=0.477, P =0.704; group: F (1,12)=0.560, P =0.469). Furthermore, the effect of DCS on active lever responding (one-way ANOVA, P <0.007, using Bonferroni correction) was observed on days 2, 5 and 8 only. The groups did not differ during training or extinction, receiving both similar total numbers of light–food pairings (Saline=662.9±44.5, DCS=652.0±36.5; one-way ANOVA; F (1,12)=0.038, P =0.848) and similar numbers of non-reinforced light presentations during extinction (Saline=122.6±11.8, DCS=129.4±15.2; one-way ANOVA; F (1,12)=0.108, P =0.748). Therefore, DCS potentiated appetitive memory extinction in a quantitative manner. However, the extinguished memory recovered with repeated testing, as observed previously with more extensive extinction training [23] . Auditory fear memory Given that in the appetitive setting, reactivation+extinction results in memory impairment under parametric conditions that render the potentiative effect of DCS ineffective, we tested whether this dissociation between behavioural and pharmacological treatments extends to the aversive domain. We have previously demonstrated that DCS enhances the extinction of an auditory fear memory [24] . Therefore, we used the same parameters of fear conditioning and extinction to assess the impact of memory reactivation 1 h before extinction. The combination of memory reactivation and extinction did affect subsequent conditioned freezing compared with the control group given extinction training alone ( Fig. 4a ). However, the direction of the effect was opposite to that which would have been expected for a reactivation+extinction impairment of auditory fear memory. The decrease in freezing from the first CS presentation at reactivation/extinction to the test session was greater in the extinction group than the reactivation+extinction group (mixed ANOVA; session×condition: F (1,14)=7.105, P =0.018). One-way ANOVA revealed that although there were no absolute differences between the conditions at reactivation/extinction ( F (1,14)=1.430, P =0.252) or test ( F (1,14)=3.693, P =0.075), the extinction-alone rats reduced their freezing levels from extinction to test ( F (1,7)=14.112, P =0.007), whereas the reactivation+extinction rats did not ( F (1,7)=1.068, P =0.336). Moreover, the reduction in conditioned freezing over CS presentations during extinction was retarded in the reactivation+extinction group compared with extinction alone ( Fig. 4b ). Therefore, memory reactivation before limited extinction training impaired both the acquisition and subsequent retention of extinction. 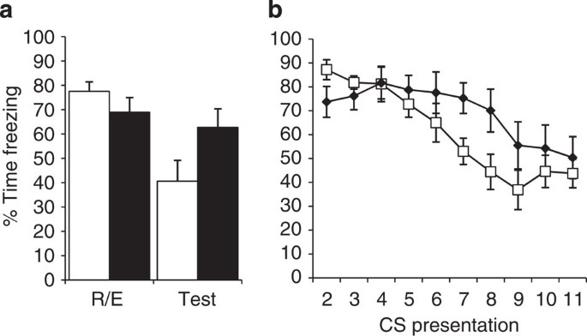Figure 4: Fear conditioning to a discrete clicker. Rats were reactivated and extinguished 1 h later (filled columns/symbols,N=8) or given extinction alone (open columns/symbols,N=8). (a) Freezing to the clicker at reactivation/start of extinction (R/E) and at the post-extinction test. Reactivation and extinction impaired the decrement in memory expression compared with extinction alone. (b) Freezing during the extinction session. The final ten presentations of the CS (that is, excluding the initial presentation of extinction or the prior reactivation presentation) are presented. The reduction in freezing levels across CS presentations was retarded in the reactivation+extinction condition, compared with the extinction alone condition (mixed ANOVA; presentation×condition:F(4.6,64.3)=3.025,P=0.019; condition:F(1,14)=1.228,P=0.286). Analysis of simple effects (P<0.05) revealed that both conditions reduced their freezing levels across the session, and there was no absolute difference between the conditions at any of the CS presentations. Data presented as mean±s.e.m. Figure 4: Fear conditioning to a discrete clicker. Rats were reactivated and extinguished 1 h later (filled columns/symbols, N =8) or given extinction alone (open columns/symbols, N =8). ( a ) Freezing to the clicker at reactivation/start of extinction (R/E) and at the post-extinction test. Reactivation and extinction impaired the decrement in memory expression compared with extinction alone. ( b ) Freezing during the extinction session. The final ten presentations of the CS (that is, excluding the initial presentation of extinction or the prior reactivation presentation) are presented. The reduction in freezing levels across CS presentations was retarded in the reactivation+extinction condition, compared with the extinction alone condition (mixed ANOVA; presentation×condition: F (4.6,64.3)=3.025, P =0.019; condition: F (1,14)=1.228, P =0.286). Analysis of simple effects ( P <0.05) revealed that both conditions reduced their freezing levels across the session, and there was no absolute difference between the conditions at any of the CS presentations. Data presented as mean±s.e.m. Full size image Contextual fear memory To disambiguate whether reactivation + extinction results in reconsolidation-mediated memory updating or a potentiation of extinction, we used the LVGCC-blocker nimodipine to prevent the reconsolidation-critical process of memory destabilization in a contextual fear memory [22] . Rats were injected with nimodipine or vehicle at differing timepoints. First, we analysed whether the combination of reactivation and extinction produced differing effects from extinction alone ( Figs 5 , 6 , 7 , 8 ; vehicle control groups). Collapsing across the timing of vehicle injection, we compared freezing during the initial post-extinction test and the post-reconditioning test for the two behavioural conditions. Whereas rats that received extinction alone significantly reacquired the contextual fear memory with a less intense footshock, those that received reactivation and extinction showed little evidence of reacquisition (mixed ANOVA; session × condition: F (1,22)=11.815, P =0.002). There were no differences between freezing levels in the two behavioural conditions at reactivation compared with the equivalent time period at the start of extinction (extinction alone=51.6±6.8, reactivation + extinction=48.4±5.4; one-way ANOVA; F (1,22)=0.108, P =0.746), indicating that there were no differences in the levels of conditioning between the groups. Moreover, simple effects analysis with separate ANOVAs revealed no group differences at the first test after reactivation and extinction ( F (1,22)=0.104, P =0.751). In contrast, rats subjected to reactivation + extinction froze significantly less than the extinction alone group at the post-reacquisition test ( F (1,22)=11.782, P =0.002). Analysis of the reactivation+extinction condition alone revealed that there was no evidence of reconditioning as the freezing levels did not differ between the two tests ( F (1,11)=3.878, P =0.075). 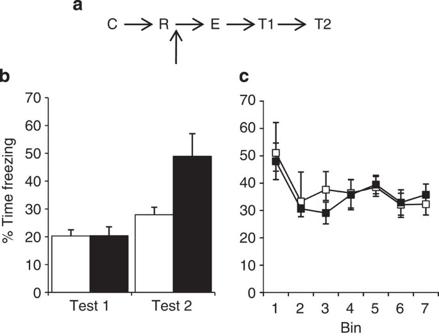Figure 5: Post-reactivation Nimodipine prevents behavioural memory updating. (a) Experimental timeline. Following contextual fear conditioning (C), Nimodipine was injected immediately after memory reactivation (R), and hence 1 h before extinction (E). (b) Subsequent freezing behaviour was compared across the post-reactivation/extinction test (T1/Test 1) and the post-reacquisition test (T2/Test 2). Nimodipine-treated rats (filled columns/symbols) readily reconditioned, whereas vehicle-treated (open columns/symbols) rats showed a persistent impairment in contextual fear. (c) Freezing during the extinction session itself did not differ between groups. Contextual freezing was compared across seven 4-min bins corresponding to the final 28 min of extinction after reactivation or the first 2 min of extinction. There were no differences between the groups during extinction (bin×treatment:F(2.0,20.5)=0.321,P=0.733; treatment:F(1,10)=0.374,P=0.554). Although there was a trend for both groups to reduce their freezing response to the context over the course of the session, this was not statistically significant (bin:F(2.0,20.5)=5.743,P=0.066). Data presented as mean+s.e.m.N=6 per group. Figure 5: Post-reactivation Nimodipine prevents behavioural memory updating. ( a ) Experimental timeline. Following contextual fear conditioning (C), Nimodipine was injected immediately after memory reactivation (R), and hence 1 h before extinction (E). ( b ) Subsequent freezing behaviour was compared across the post-reactivation/extinction test (T1/Test 1) and the post-reacquisition test (T2/Test 2). Nimodipine-treated rats (filled columns/symbols) readily reconditioned, whereas vehicle-treated (open columns/symbols) rats showed a persistent impairment in contextual fear. ( c ) Freezing during the extinction session itself did not differ between groups. Contextual freezing was compared across seven 4-min bins corresponding to the final 28 min of extinction after reactivation or the first 2 min of extinction. There were no differences between the groups during extinction (bin×treatment: F (2.0,20.5)=0.321, P =0.733; treatment: F (1,10)=0.374, P =0.554). Although there was a trend for both groups to reduce their freezing response to the context over the course of the session, this was not statistically significant (bin: F (2.0,20.5)=5.743, P =0.066). Data presented as mean+s.e.m. N =6 per group. 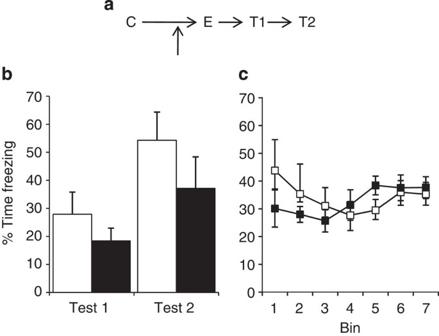Figure 6: Pre-extinction Nimodipine has no effect on memory extinction. (a) Experimental timeline. Following contextual fear conditioning (C), Nimodipine was injected 1 h before extinction (E). (b) Subsequent freezing behaviour was compared across the post-reactivation/extinction test (T1/Test 1) and the post-reacquisition test (T2/Test 2). Both vehicle- (open columns/symbols) and Nimodipine-treated (filled columns/symbols) rats readily reconditioned. (c) Freezing during the extinction session itself did not differ between groups. Contextual freezing was compared across seven 4-min bins corresponding to the final 28 min of extinction after reactivation or the first 2 min of extinction. There were no differences between the groups during extinction (bin×treatment:F(2.2,22.1)=2.038,P=0.150; treatment:F(1,10)=0.020,P=0.889). However, there was also no evidence for a reduction of freezing over the course of the session (bin:F(2.2,22.1)=1.762,P=0.193). Data presented as mean+s.e.m.N=6 per group. Full size image Figure 6: Pre-extinction Nimodipine has no effect on memory extinction. ( a ) Experimental timeline. Following contextual fear conditioning (C), Nimodipine was injected 1 h before extinction (E). ( b ) Subsequent freezing behaviour was compared across the post-reactivation/extinction test (T1/Test 1) and the post-reacquisition test (T2/Test 2). Both vehicle- (open columns/symbols) and Nimodipine-treated (filled columns/symbols) rats readily reconditioned. ( c ) Freezing during the extinction session itself did not differ between groups. Contextual freezing was compared across seven 4-min bins corresponding to the final 28 min of extinction after reactivation or the first 2 min of extinction. There were no differences between the groups during extinction (bin×treatment: F (2.2,22.1)=2.038, P =0.150; treatment: F (1,10)=0.020, P =0.889). However, there was also no evidence for a reduction of freezing over the course of the session (bin: F (2.2,22.1)=1.762, P =0.193). Data presented as mean+s.e.m. N =6 per group. 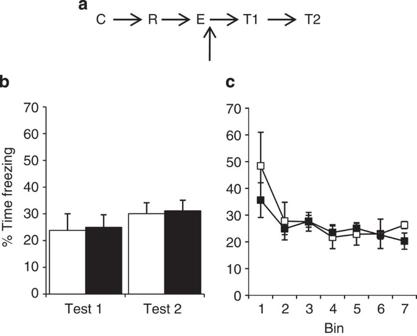Figure 7: Post-extinction Nimodipine has no effect on behavioural memory updating. (a) Experimental timeline. Following contextual fear conditioning (C) and memory reactivation (R), Nimodipine was injected immediately after extinction (E). (b) Subsequent freezing behaviour was compared across the post-reactivation/extinction test (T1/Test 1) and the post-reacquisition test (T2/Test 2). Both vehicle- (open columns/symbols) and Nimodipine-treated (filled columns/symbols) rats failed to recondition. (c) Freezing during the extinction session itself did not differ between groups. Contextual freezing was compared across seven 4-min bins corresponding to the final 28 min of extinction after reactivation or the first 2 min of extinction. There were no differences between the groups during extinction (bin x treatment:F(1.6,15.8)=0.858,P=0.418; treatment:F(1,10)=0.342,P=0.572). Both groups extinguished their freezing response to the context over the course of the session (bin:F(1.6,15.8)=5.743,P=0.018). Data presented as mean+s.e.m.N=6 per group. Full size image Figure 7: Post-extinction Nimodipine has no effect on behavioural memory updating. ( a ) Experimental timeline. Following contextual fear conditioning (C) and memory reactivation (R), Nimodipine was injected immediately after extinction (E). ( b ) Subsequent freezing behaviour was compared across the post-reactivation/extinction test (T1/Test 1) and the post-reacquisition test (T2/Test 2). Both vehicle- (open columns/symbols) and Nimodipine-treated (filled columns/symbols) rats failed to recondition. ( c ) Freezing during the extinction session itself did not differ between groups. Contextual freezing was compared across seven 4-min bins corresponding to the final 28 min of extinction after reactivation or the first 2 min of extinction. There were no differences between the groups during extinction (bin x treatment: F (1.6,15.8)=0.858, P =0.418; treatment: F (1,10)=0.342, P =0.572). Both groups extinguished their freezing response to the context over the course of the session (bin: F (1.6,15.8)=5.743, P =0.018). Data presented as mean+s.e.m. N =6 per group. 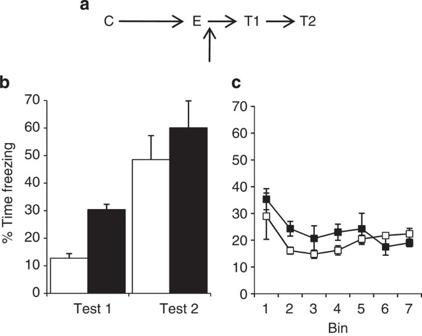Figure 8: Post-extinction Nimodipine impairs memory extinction. (a) Experimental timeline. Following contextual fear conditioning (C), Nimodipine was injected after extinction (E). (b) Subsequent freezing behaviour was compared across the post-reactivation/extinction test (T1/Test 1) and the post-reacquisition test (T2/Test 2). Nimodipine-treated rats (filled columns/symbols) were impaired compared with vehicle-treated controls (open columns/symbols) in extinction retention at Test 1. (c) Freezing during the extinction session itself did not differ between groups. Contextual freezing was compared across seven 4-min bins corresponding to the final 28 min of extinction after reactivation or the first 2 min of extinction. There were no differences between the groups during extinction (bin x treatment:F(2.4,24.1)=1.421,P=0.262; treatment:F(1,10)=1.608,P=0.234). Both groups showed extinguished their freezing response to the context over the course of the session (bin:F(2.4,24.1)=5.078,P=0.011) Data presented as mean+s.e.m.N=6 per group. Full size image Figure 8: Post-extinction Nimodipine impairs memory extinction. ( a ) Experimental timeline. Following contextual fear conditioning (C), Nimodipine was injected after extinction (E). ( b ) Subsequent freezing behaviour was compared across the post-reactivation/extinction test (T1/Test 1) and the post-reacquisition test (T2/Test 2). Nimodipine-treated rats (filled columns/symbols) were impaired compared with vehicle-treated controls (open columns/symbols) in extinction retention at Test 1. ( c ) Freezing during the extinction session itself did not differ between groups. Contextual freezing was compared across seven 4-min bins corresponding to the final 28 min of extinction after reactivation or the first 2 min of extinction. There were no differences between the groups during extinction (bin x treatment: F (2.4,24.1)=1.421, P =0.262; treatment: F (1,10)=1.608, P =0.234). Both groups showed extinguished their freezing response to the context over the course of the session (bin: F (2.4,24.1)=5.078, P =0.011) Data presented as mean+s.e.m. N =6 per group. Full size image When nimodipine (16 mg kg −1 ) was injected immediately after memory reactivation, and hence 60 min before the subsequent extinction training, there was a significant disruption of the reactivation+extinction effect on fear relearning ( Fig. 5a ; mixed ANOVA; session × treatment: F (1,10)=11.004, P =0.008; treatment: F (1,10)=4.148, P =0.069). The groups did not differ in the levels of contextual fear acquired before treatment (vehicle=52.4±11.2, nimodipine=46.9±5.7; one-way ANOVA; F (1,10)=0.229, P =0.643), or during the course of extinction training ( Fig. 5b ). Moreover, analysis of simple effects with separate ANOVAs revealed that although there was no effect of nimodipine on freezing at the post-reactivation +extinction test ( F (1,10)=0.001, P =0.975), the nimodipine-treated group froze significantly more at the post-reacquisition test ( F (1,10)=7.247, P =0.023). In contrast, injection of nimodipine 60 min before extinction in the extinction-alone condition had no effect on post-extinction contextual freezing, with both the nimodipine and vehicle groups successfully reacquiring the contextual fear memory to a similar degree ( Fig. 6a ; mixed ANOVA; session × treatment: F (1,10)=0.382, P =0.550; treatment: F (1,10)=1.517, P =0.246; session: F (1,10)=13.388, P =0.004). Although the rats treated with nimodipine were impaired in the levels of freezing in the first 2 min of extinction (vehicle=64.9±8.7, nimodipine=31.9±8.6; one-way ANOVA; F (1,10)=7.284, P =0.022), they were not impaired in either the acquisition ( Fig. 6b ) or retention of memory extinction. When nimodipine was injected immediately after the extinction phase in the reactivation+extinction condition, it produced no effect on subsequent contextual freezing and fear memory reacquisition ( Fig. 7a ; mixed ANOVA; session × treatment: F (1,10)=0.000, P =0.994; treatment: F (1,10)=0.062, P =0.808). A lack of main effect of session ( F (1,10)=2.122, P =0.176) revealed that neither group showed an increase in freezing after reacquisition. There were no group differences at memory reactivation (vehicle=44.4±7.6, nimodipine=46.5±7.6; one-way ANOVA; F (1,10)=0.047, P =0.833). Moreover, there was no difference between the groups during extinction training itself ( Fig. 7b ). Therefore, nimodipine had no impact on the effect of reactivation+extinction to disrupt the contextual fear memory. In contrast, nimodipine injection immediately after extinction training impaired the extinction memory ( Fig. 8a ; mixed ANOVA; session × treatment: F (1,10)=0.275, P =0.611; treatment: F (1,10)=5.067, P =0.048). Given that an impairment in memory extinction would be expected to be most apparent in the post-extinction test, planned one-way ANOVAs analysed the two tests separately. Nimodipine-treated rats froze significantly more than vehicle-treated controls at the post-extinction test ( F (1,10)=58.133, P <0.001), but not at the post-reacquisition test ( F (1,10)=0.904, P =0.364). There were also no differences between the groups at the start of extinction training, indicating that the differences thereafter were not attributable to pre-existing differences in the level of conditioning (vehicle=38.3±11.2, nimodipine=42.6±4.8; F (1,10)=0.154, P =0.703). Moreover, there was no difference between the groups during extinction training itself ( Fig. 8b ). The combination of memory reactivation followed 1 h later by extinction training resulted in a persistent memory impairment in two settings. Firstly, the appetitive pavlovian memory mediating conditioned reinforcement was diminished through several days of testing and reinstatement. Secondly, a contextual fear memory was impaired to the extent that reacquisition was retarded. These effects of reactivation and extinction seem to be mediated by a behavioural updating of the reconsolidation process, rather than a potentiation of extinction. Memory reconsolidation of sucrose–associated memories in a conditioned reinforcement setting has previously been disrupted by NMDA receptor antagonism using a 10-min reactivation session [6] . This suggests that the light–food memory in the present study was functionally reactivated by the 10-min reactivation, engaging the reconsolidation process. Adding the extinction training 1 h later resulted in memory impairment that neither recovered with repeated testing, nor reinstated with pre-test exposure to the food outcome. By contrast, increasing the interval between reactivation and extinction to 6 h resulted in little evidence of memory impairment. Context re-exposure for 10 min was equally effective in reactivating the appetitive pavlovian memory. The context re-exposure condition has been used as the control for fear conditioning [9] but is clearly inappropriate in the current appetitive setting. The efficacy of context exposure to reactivate memories is mixed. We have previously observed that context exposure does not successfully reactivate a strongly learned light–cocaine memory, at least as assessed by the amnestic impact of intra-amygdala infusions of Zif268 antisense oligodeoxynucleotides [17] . However, in human episodic memories, context seems to be the single most important trigger for memories to undergo reconsolidation [25] . Therefore, the capacity of context exposure to reactivate and destabilize a related discrete memory appears to be variable. Further investigation of this issue will be important, especially, given the finding that reconsolidation-based impairments are restricted to the stimulus that is presented at reactivation [26] , as effective context-mediated reactivation of discrete memories might be particularly useful in targeting sets of stimuli that are important in maintaining maladaptive behaviour. In contrast to the successful diminishing of appetitive CS–unconditioned stimulus (US) representations, the combination of reactivation and extinction did not reduce subsequent auditory conditioned freezing. Rather, it seemed to retard or impair extinction relative to an extinction-alone condition. Although this observation is in marked contrast to the original demonstration by Monfils et al . [9] , two important points must be noted. First, prior attempts to replicate the findings of Monfils et al . [9] have yielded contrasting results, with success in mice [11] , but not in an extensive examination in rats [12] . Therefore, the conditions under which auditory fear memories can be diminished through reactivation and extinction are poorly understood. Second, the extent of extinction training employed in the present study was intentionally limited to replicate the conditions under which DCS potentiates fear memory extinction [24] . The 10–11 unreinforced CS presentations differs substantially from the 18–19 used by Monfils et al . [9] Therefore, it is possible that the extent of cued fear extinction training was insufficient to observe the expected effect in the present study. This contrasts with the seemingly more robust extinction training in our contextual fear experiment, which successfully yielded a reactivation+extinction effect. Although it is tempting to characterize the reactivation and extinction impairment as a behavioural updating of the reactivated and reconsolidating memory, the pattern of results is equally consistent with a quantitative and qualitative potentiation of memory extinction, as previously achieved using DCS and fibroblast growth factor 2 (refs 19 , 20 , 21 ). However, we now have 3 lines of evidence favouring the reconsolidation-based interpretation. First, injecting DCS rather than reactivating the memory before appetitive pavlovian extinction training did not affect the subsequent acquisition of a new response with conditioned reinforcement. DCS was able to potentiate appetitive memory extinction, supporting prior observations in other appetitive memory settings [27] , [28] , [29] , but only when the extinction session was 3 hr long. Moreover, the DCS-induced potentiation of extinction resulted only in a transient deficit in conditioned reinforcement. This spontaneous recovery of the appetitive memory is in marked contrast with the persistent deficit observed following reactivation + extinction. Secondly, for cued fear memories, memory reactivation 1 h before extinction training and DCS injection in conjunction with the same extinction training produce different effects. This parametric difference between the reactivation + extinction impairment and pharmacological enhancement of extinction is consistent with the interpretation that they are mediated by qualitatively different processes. Finally, we showed that preventing memory reactivation impaired the reactivation + extinction effect in a contextual fear setting. Using a procedure known to elicit contextual fear memory reconsolidation [30] , the addition of extinction training 1 h after memory reactivation seemingly erased the contextual fear memory. This was evidenced by the reduction in freezing levels following reconditioning. Rats that were just extinguished showed high levels of post-reacquisition freezing, likely reflecting a combination of reinstatement of the extinguished memory and the effect of further conditioning. In contrast, rats given reactivation and extinction showed little evidence of reconditioning. This indicates that the original excitatory memory was impaired to the extent that reinstatement was ineffective. Moreover, the failure to recondition suggests that reactivation and extinction may in fact lead to the formation of a memory that the previously fear conditioned context is now safe [9] . LVGCCs are important not only for memory reactivation, but also for the extinction of contextual fear memories [22] . To disambiguate the effects of the LVGCC blocker nimodipine on memory reactivation and extinction, we administered it after both reactivation and extinction in separate experiments. Nimodipine impaired extinction when given immediately after extinction alone, exactly as previously demonstrated [22] . In the reactivation + extinction condition, nimodipine was without effect when administered immediately after the extinction phase. When nimodipine was injected 1 hr before extinction it had no effect on the extinction memory itself, although it did acutely impair memory retrieval. Whereas the acute effect of nimodipine is consistent with some [31] , but not all [32] , studies of LVGCCs, the lack of long-term effect on extinction memory suggests that the injection took place too far in advance to impact on extinction learning and consolidation. It has previously been observed that nimodipine injection 20 min before extinction is effective at impairing extinction retention 1 day later [32] . However, the alternative antagonist nifedipine has been shown to impair extinction when administered at each of several timepoints up to 4 h before extinction training [31] , [33] . Therefore, a full timecourse analysis of the effects of nimodipine would be required to determine the window of vulnerability of contextual fear memory extinction to nimodipine. In contrast to the lack of effect on extinction alone, nimodipine treatment immediately after memory reactivation, and hence also 60 min before the extinction phase, prevented the behavioural memory impairment characteristic of reactivation and extinction. These effects of nimodipine on post-extinction contextual freezing were not attributable to any differences in extinction learning, as there were no treatment effects on within-session freezing levels during the extinction sessions themselves. Therefore, the impact of nimodipine was most likely mediated by its effects on extinction consolidation and memory destabilisation. The divergent impact of nimodipine depending on the behavioural condition strongly suggests that its effect when given post-reactivation are due to the disruption of memory destabilisation, thereby preventing the later extinction training from behaviourally updating the memory. This means also that the reason nimodipine fails to have an effect when given immediately after the extinction phase of reactivation + extinction is that the contextual fear memory has already been destabilized, and the resultant behavioural updating through non-reinforced context exposure to disrupt the fear memory does not depend on LVGCC-based mechanisms. This interpretation based on the dissociable patterns of impairment holds regardless of the true nature of the nimodipine-induced impairment of extinction [34] . Therefore, the persistent amnestic effect of reactivation and extinction seems to be truly mediated by a behavioural hijacking of the reconsolidation process. In summary, the present results demonstrate that the memory-impairing impact of reactivation followed by extinction is applicable to appetitive discrete pavlovian memories, as well as aversive contextual fear memories. These effects represent a behavioural method of reconsolidation impairment that utilizes the memory-updating function of memory reconsolidation [2] . Moreover, given that the likely locus of effect of systemically applied nimodipine is the hippocampus [22] , these results suggest that reactivation+extinction impacts on memory mechanisms in the hippocampus as well as in the amygdala [11] . However, given that the previous demonstrations of persistent cued fear memory disruption with reactivation and extinction [9] , [10] , [11] have seemingly failed to be reproduced in a translationally relevant setting [13] , it remains to be determined whether the present disruption of pavlovian appetitive food memories will generalize to situations of addictive drug and high-incentive food seeking. Subjects The subjects were 180 experimentally naive adult male Lister Hooded rats, weighing 200–225 g at the start of the experiments. They were housed in groups of 4, in a holding room maintained at 21°C on a normal light cycle (12 h light: 12 h dark; lights on at 0700). All rats were given free access to water. Those tested on the appetitive conditioned reinforcement procedure were given restricted access to food (15 g chow per day). Rats that were fear conditioned had free access to food. All procedures were conducted in accordance with the United Kingdom 1986 Animals (Scientific Procedures) Act (PPL 40/3205). Drug administration DCS and Nimodipine were both injected intra-peritoneally. DCS was dissolved in saline (15 mg kg −1 ; 1 mg ml −1 ). This dose was effective in potentiating the extinction of fear and drug-associated memories [19] , [24] , [28] , [35] . Nimodipine (16 mg kg −1 ) was sonicated into 100% Cremophor EL and then diluted to a concentration of 8 mg ml −1 in a final vehicle of 10% Cremophor and 2.5% dimethylsulphoxide in saline with 1 drop Tween 80 per 3 ml. This dose has previously been demonstrated to impair both the reactivation and extinction of contextual fear memories [22] , [32] . Behavioural apparatus The rats were trained and tested in eight operant chambers (MedAssociates) as previously described [36] . Each chamber had a nosepoke magazine attached to a pellet dispenser, as well as two retractable levers with a stimulus light located above each one. In addition, four of the chambers, used for the fear-conditioning experiments, were fitted with clicker modules, shock generators and scramblers, and infra-red video cameras (Viewpoint Life Sciences). Behavioural procedures Conditioned reinforcement: in 9 days of appetitive memory acquisition, the rats were trained to nosepoke into the magazine to receive a food pellet (45 mg grain-based reward pellet; TestDiet). The delivery of the food pellet was associated with illumination of one of the stimulus lights (right or left, counterbalanced) and extinction of the houselight for 10 s. During this 10-s period, further nosepokes were recorded, but had no programmed consequence. The training sessions lasted 20 min and there was no limit to the number of pellets that could be earned in each session. One group of rats received 2 sessions of context pre-exposure before training began. These sessions were 90-min long on each day, and rats could nosepoke, but there was no programmed consequence. In the day after the final training session, the reactivation and extinction procedures were conducted. Memory reactivation consisted of a 10-min extinction session, in which nosepoke responses were reinforced by the light stimulus, but no pellets were delivered. Extinction was operationally identical, but in a longer session of 60 or 70 min (the latter as the control for total reactivation+extinction time). Groups of rats that were given a context exposure instead of memory reactivation were returned to the operant chambers for 10 min, but nosepokes had no programmed consequence. A final group was subjected to the context exposure, but a transparent Perspex sheet was placed in front of the wall containing the nosepoke magazine and light stimuli to prevent the rats from performing the nosepoke response. The rats were returned to their homecages in between reactivation and extinction. For the DCS experiments, there was no memory reactivation or context exposure, and DCS or saline was injected 30 min before a 60-min or 180-min extinction session. The testing phase involved the extension of the levers into the chambers for the first time. A response on the active lever on the opposite side to the light stimulus resulted in illumination of the light as a conditioned reinforcer. A response on the inactive lever below the location of the light stimulus, or a nosepoke response, had no programmed consequence. Discriminated responding on the active lever over and above responding on the inactive lever, over several days of testing is a sensitive measure of the acquired conditioned reinforcing properties of appetitive pavlovian stimuli. The test sessions were 30-min long, and were conducted on 6 occasions over a period of 20 days. For the first four sessions, the active lever response was reinforced by the light stimulus under an FR1 schedule. The schedule was increased to FR1-3 for the remaining sessions to increase response output and thereby promote the possibility of spontaneous recovery. A final reinstatement test was conducted 7 days after the last test. This session was preceded by a 5-min context exposure, during which the rats were allowed to retrieve and consume 10 pellets that were freely available, to test for outcome-induced reinstatement of the diminished memory. Auditory fear conditioning: Rats were first habituated to the operant chambers for 2 h on the day before conditioning. For fear conditioning, the rats were again placed in the operant chambers, and after a 30-min habituation period, were subjected to two CS–US pairings with an intertrial interval of 5 min. The CS was an auditory clicker (10 Hz, 80 dB, 60 s) and the US was a mild electric footshock (0.5 mA, 0.5 s). On the day after fear conditioning, the rats were first subjected to a 2-min memory reactivation session, in which the 60-s CS was presented after 60 s. One hour later, the rats received a 20-min extinction session, involving 10 CS presentations with an interstimulus interval of 60 s. The control group received a single 22-min extinction session with 11 CS presentations. No footshocks were delivered in any of the reactivation or extinction sessions. On the next day, the final fear memory test was undertaken, consisting of a single presentation of the 60-s CS after 60 s in a 2-min session. Freezing behaviour was automatically scored throughout all the sessions using Videotrack software (Viewpoint Life Sciences). Contextual fear conditioning: for fear conditioning, the rats were placed into the operant chambers for 3 min, and after 2 min a single footshock (0.5 mA, 2 s) was delivered. On the next day, the contextual fear memory was reactivated by returning the rats to the chamber for 2 min. One hour later, the rats received a 28-min extinction session in the same context. Extinction-alone controls received a single 30-min extinction session. The next day, all rats were tested for contextual fear memory and were also reconditioned using a less intense footshock (0.35 mA, 2 s) to test for savings. This took place in a single 3-min conditioning session, with the initial 2 min exposure serving as the test period, at the end of which the footshock was delivered. Finally, there was a 2-min post-reconditioning test on day 4. The rats were injected with Nimodipine (16 mg kg −1 ) or vehicle either immediately after the extinction phase, or immediately after reactivation/60 min before extinction. Statistical analysis The appetitive data were analysed using mixed factorial ANOVA with factors lever (active versus inactive), session (days of testing) and group (behavioural condition) as appropriate. The data were checked for normality, using the Shapiro–Wilk test. The Greenhouse–Geisser correction was employed in all analyses as the assumption of sphericity was always violated. Analysis of the training, reactivation and extinction data consisted of individual one-way ANOVAs on the total number of light–food pairings and the numbers of non-reinforced light presentations across groups. For the freezing data, the % time freezing was analysed using mixed factorial ANOVA with factors session, behavioural condition and treatment (nimodipine versus vehicle) as appropriate. As the anticipated effects of nimodipine were expected to differ between the two test sessions, planned comparisons for the effect of treatment at each test were carried out. A significance level of P <0.05 was used for all analyses. How to cite this article: Flavell, C.R. et al . Behavioural memory reconsolidation of food and fear memories. Nat. Commun. 2:504 doi: 10.1038/ncomms1515 (2011).